A high-rate long-life Li4Ti5O12/Li[Ni0.45Co0.1Mn1.45]O4lithium-ion battery Lithium batteries are receiving considerable attention as storage devices in the renewable energy and sustainable road transport fields. However, low-cost, long-life lithium batteries with higher energy densities are required to facilitate practical application. Here we report a lithium-ion battery that can be cycled at rates as high as 10 C has a life exceeding 500 cycles and an operating temperature range extending from −20 to 55 °C. The estimated energy density is 260 W h kg −1 , which is considerably higher than densities delivered by the presently available Li-ion batteries. The replacement of internal combustion engine cars with electric vehicles, such as hybrid vehicles, plug-in hybrid vehicles and, ultimately, full electric vehicles, will require the development of advanced rechargeable batteries. Li-ion batteries have high intrinsic energy density values and are promising candidates [1] , [2] , but current Li-ion battery technologies are not yet able to meet the requirements of efficiently storing alternative energy sources and/or powering hybrid or electric vehicles. Reduction in cost, enhancement in safety, and improvement in energy density are the main properties that have to be implemented. To achieve these important goals, a renewal in the present lithium battery chemistry, aimed at the replacement of costly and unsafe lithium cobalt oxide and of thermodynamically unstable graphite with alternative, morphologically upgraded, reliable cathode and anode, respectively, is mandatory [3] , [4] , [5] . Here we report a high-performance lithium-ion battery that exploits a unique electrode combination. The battery utilizes existing concepts but offers performances that, to our knowledge, have never been met by other systems. We show that the battery can be cycled at rates as high as 10 C rate with minor decays in capacity, that it has an unusually long life: exceeding 500 cycles at 1 C rate; and may operate over a wide temperature range: from −20 °C to 55 °C, with no substantial losses in cycling stability and capacity delivery. Battery structure The battery developed in this work is based on the combination of a Li 4 Ti 5 O 12 (LTO) negative electrode with a Li[Ni 0.45 Co 0.1 Mn 1.45 ]O 4 (LNMO)-positive electrode. LTO is a well-known material benefitting by a series of important properties when exploited as electrode in lithium cells, including: minor or no volume changes during cycling and voltage excursion comprised within the electrochemical windows of most common electrolytes [6] , [7] , [8] , [9] . Accordingly, LTO may be repeatedly cycled without inducing any electrolyte decomposition [10] , [11] . However, these favourable aspects may be contrasted by relatively low rates, unless LTO is prepared with adequate, specially designed morphology. Advanced LTO electrode By a synthesis procedure originally conceived in our laboratory [12] , we have developed a C-coated microscale LTO involving composites between nano-sized LTO particles and carbon. 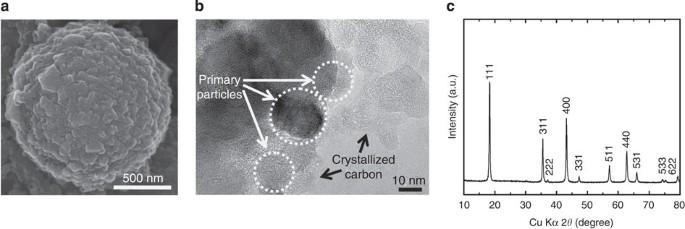Figure 1: Morphological and structural analysis of LTO. (a) Reports a scanning electron microscopy image of the LTO particles showing that they are formed by aggregates of nano-sized LTO particles. (b) Shows the TEM images of the powder material revealing that the LTO particles are intimately interconnected by carbon bridges. (c) The X-ray diffraction pattern of the LTO, revealing the occurrence of all the peaks associated with LTO, so demonstrating the purity of the material and confirming the nano-size of its primary particles as evidenced by the TEM analysis. This particular morphology is clearly shown by the scanning electron microscopy and transmission electron microscopy (TEM) images reported in Figure 1 . Figure 1a shows that that the aggregates of nano-sized LTO particles and Figure 1b that these particles are intimately interconnected by carbon bridges. The X-ray diffraction, also included in the same Figure 1 , reveals the occurrence of all the peaks associated with LTO, so demonstrating the purity of the material and confirming the nano-size of its primary particles as evidenced by the TEM analysis. Figure 1: Morphological and structural analysis of LTO. ( a ) Reports a scanning electron microscopy image of the LTO particles showing that they are formed by aggregates of nano-sized LTO particles. ( b ) Shows the TEM images of the powder material revealing that the LTO particles are intimately interconnected by carbon bridges. ( c ) The X-ray diffraction pattern of the LTO, revealing the occurrence of all the peaks associated with LTO, so demonstrating the purity of the material and confirming the nano-size of its primary particles as evidenced by the TEM analysis. Full size image The carbon bridges act as electron pathways that electrically interconnect the LTO particles, ultimately providing the electrode with a very high conductivity that, combined with the reduction of the lithium diffusion length within the particles (10–20 nm in diameter, see TEM image of Fig. 1 ), is expected to provide the LTO electrode with fast kinetics. 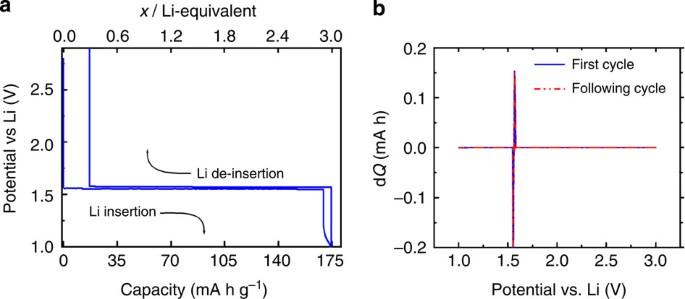Figure 2: Electrochemical characterization of LTO. (a) Shows the voltage profile of the first charge (lithium acceptance)-discharge (lithium removal) cycle of a C-LTO composite electrode in a lithium cell. The voltage evolves over the expected 1.5 V with almost no polarization between charge and discharge and with a capacity delivery approaching the theoretical 175 mAh g−1value. (b) Reports the incremental charge (dQ) versus potential curve of the PCGA analysis of two consecutive cycles of the C-LTO composite electrode in a lithium cell. The traces overlap with almost no separation between anodic and cathodic peaks. Room temperature. This is indeed confirmed by Figure 2 that shows the voltage profile of the first charge (lithium acceptance)–discharge (lithium removal) cycle (a) and incremental charge (d Q ) versus potential (b) curve of the potentiodynamic cycling with galvanostatic acceleration (PCGA) analysis of two consecutive cycles of the C-coated LTO electrode in a lithium cell. The PCGA analysis is a quasi-equilibrium technique that can provide very useful detailed information of the characteristics of electrochemical processes [13] . We see from Figure 2b that the electrode cycles along the expected plateau at about 1.5 V versus Li/Li + , with a capacity delivery approaching the theoretical value of 175 mA h g −1 . Most impressive is the absence of hysteresis between charge and discharge profiles, an effect that indicates a very high coulombic efficiency and very fast kinetics. Figure 2b , reporting the incremental charge d Q versus potential extended for two consecutive cycles, evidences that the traces overlap and there is almost no separation between the anodic and the cathodic peaks. All the above evidences provide convincing proofs of the excellent cycle life and rate capability of our C-coated LTO electrode. Figure 2: Electrochemical characterization of LTO. ( a ) Shows the voltage profile of the first charge (lithium acceptance)-discharge (lithium removal) cycle of a C-LTO composite electrode in a lithium cell. The voltage evolves over the expected 1.5 V with almost no polarization between charge and discharge and with a capacity delivery approaching the theoretical 175 mAh g −1 value. ( b ) Reports the incremental charge (dQ) versus potential curve of the PCGA analysis of two consecutive cycles of the C-LTO composite electrode in a lithium cell. The traces overlap with almost no separation between anodic and cathodic peaks. Room temperature. 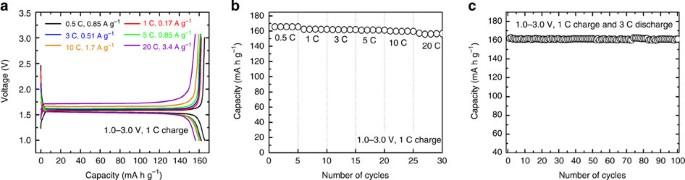Figure 3: Performance of the C-LTO electrode in a lithium cell. (a) Illustrates the voltage profiles of the C-LTO electrode cycled at various rates, showing that the electrode can be effectively cycled at current rates as high as 20C rate while still maintaining a capacity delivery of 156 mAh g−1, that is 89% of the maximum, theoretical value (b). (c) Shows that the high delivered capacity of 162 mAh g−1can be maintained without any evidence of decay for over 100 cycles run at 3C rate. Room temperature. Full size image This conclusion is further supported by Figure 3 that summarizes the response of the electrode in a lithium cell. The data demonstrate that the electrode can be effectively cycled at current rates as high as 20 C rate while still maintaining a capacity delivery of 156 mA h g −1 , that is 89% of the maximum, theoretical value ( Fig. 3a ) and that the delivered capacity of 162 mAh g −1 at 3 C rate can be maintained without any evidence of decay for over 100 cycles ( Fig. 3c ). We are not aware of other micro-sized LTO electrodes capable of meeting these performances. Finally, it has to be noticed that a key parameter for an electrode to be used in practical batteries is the value of the tap density that in turn reflects the volumetric energy density of the battery. The common approach to achieve high volumetric capacity is to prepare the LTO electrode in micro-size, spherical, and dense particles. However, while having a high tap density, these micro-size LTO electrodes usually suffer from poor capacity and rate capability, because of the limitation induced by the long Li + diffusion path throughout the particles [14] , [15] . On the contrary, our LTO electrode, in virtue of its unique nanoporous morphology exploiting a uniform, highly conductive carbon-coating layer, marks superiority over conventional materials, by offering a relatively high tap density, that is, 1.31 g cm −3 combined with excellent electrochemical performance. Figure 3: Performance of the C-LTO electrode in a lithium cell. ( a ) Illustrates the voltage profiles of the C-LTO electrode cycled at various rates, showing that the electrode can be effectively cycled at current rates as high as 20C rate while still maintaining a capacity delivery of 156 mAh g −1 , that is 89% of the maximum, theoretical value ( b ). ( c ) Shows that the high delivered capacity of 162 mAh g −1 can be maintained without any evidence of decay for over 100 cycles run at 3C rate. Room temperature. Full size image The positive electrode material The cathode selected for combination with LTO is the LNMO spinel. The preparation of this material is also based on a synthesis originally developed in our laboratory. Its basic characteristics in a lithium cell have been reported in a previous work [16] . For a matter of consistency, that is, to check whether the response of the LNMO electrode matches that of LTO, we only report here the voltage profiles and the differential capacity (d Q /d V ) curves in a lithium cell. 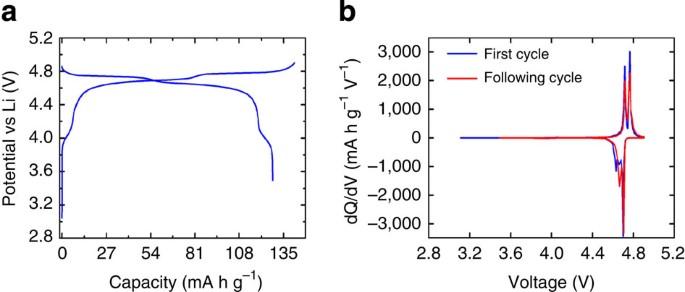Figure 4: Performance of the LNMO electrode in a lithium cell. (a) Illustrates the voltage profiles of the LNMO electrode cycled at 0.2C (A). The Figure clearly shows that the LNMO electrode operates with two subsequent plateaus, corresponding to the two redox processes of nickel, that is Ni2+/Ni3+and Ni3+/Ni4+, at 4.6 V and 4.7 V, versus Li, respectively. The two steps are clearly evidenced in the corresponding derivative dQ/dV response shown in (b): the overlap of the peaks and their very small separation suggest that this electrode operates with a high efficiency, a long cycling life and fast kinetics. Room temperature. Figure 4 shows that the LNMO electrode operates with two plateaus, corresponding to the two redox processes of nickel, that is, Ni 2+ /Ni 3+ and Ni 3+ /Ni 4+ , at 4.6 V and 4.7 V, respectively. The two steps are clearly evidenced in the corresponding d Q /d V response: the overlap of the peaks and their very small separation suggest that also this electrode operates with a high efficiency, a long cycling life and fast kinetics. The tap density of the LNMO electrode is 2.20 g cm −3 , a value that compares well with that of LTO. Figure 4: Performance of the LNMO electrode in a lithium cell. ( a ) Illustrates the voltage profiles of the LNMO electrode cycled at 0.2C (A). The Figure clearly shows that the LNMO electrode operates with two subsequent plateaus, corresponding to the two redox processes of nickel, that is Ni 2+ /Ni 3+ and Ni 3+ /Ni 4+ , at 4.6 V and 4.7 V, versus Li, respectively. The two steps are clearly evidenced in the corresponding derivative dQ/dV response shown in ( b ): the overlap of the peaks and their very small separation suggest that this electrode operates with a high efficiency, a long cycling life and fast kinetics. Room temperature. Full size image The Li[Ni 0.45 Co 0.1 Mn 1.45 ]O 4 electrode material discussed here differs from the more conventional Li[Ni 1/2 Mn 3/2 ]O 4 (refs 17 , 18 ) for the unique role of the Co substitution for both Ni and Mn, thus improving structural stability and electronic conductivity, finally resulting in an electrode having high cycling stability and rate capability. As expected from their respective voltages, the combination of LTO with LNMO gives rise to a battery operating in the 3 V range. 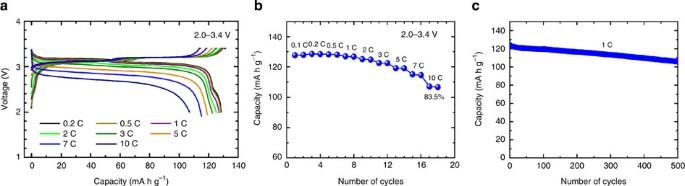Figure 5: Performance of the LTO/LNMO battery at various rates. (a) Shows the voltage profiles of the charge (lithium transfer from LNMO to LTO)-discharge (back transfer of lithium from LTO to LNMO) cycles of the battery run at various rates. As expected from their respective voltages, the combination of LTO with LNMO gives rise to a battery operating in the 3 V range. (b) Reports the capacity delivery at increasing rate regimes demonstrating that at rates as high as 10 C still 83.5% of the initial capacity is provided by the battery. (c) Shows that the battery may sustain a life extending to 500 cycles with only 14.6% capacity loss. Room temperature. Figure 5a shows the voltage profiles of the charge (lithium transfer from LNMO to LTO)–discharge (back transfer of lithium from LTO to LNMO) cycles of the battery. To be noticed that both the very flat voltage profile centered on 3 V and the very small hysteresis between charge and discharge behavior during a long cycling effect are concrete evidences of high reversibility and fast kinetics. The battery, in fact, may be cycled at 1 C rate with 128 mA h g −1 capacity delivery, that is, at a value closed to the theoretical one (the battery is cathode limited) ( Fig. 5a ) and for a life extending 500 cycles with only 14.6% capacity loss, ( Fig. 5c ). Also, the battery has excellent rate performance and can be cycled up to 10 C with the only 16.5% capacity decay ( Fig. 5c ). Figure 5: Performance of the LTO/LNMO battery at various rates. ( a ) Shows the voltage profiles of the charge (lithium transfer from LNMO to LTO)-discharge (back transfer of lithium from LTO to LNMO) cycles of the battery run at various rates. As expected from their respective voltages, the combination of LTO with LNMO gives rise to a battery operating in the 3 V range. ( b ) Reports the capacity delivery at increasing rate regimes demonstrating that at rates as high as 10 C still 83.5% of the initial capacity is provided by the battery. ( c ) Shows that the battery may sustain a life extending to 500 cycles with only 14.6% capacity loss. Room temperature. Full size image Finally, a crucial parameter for a battery addressed to the storage of renewable energy sources, as well as to the powering of electric car engines, is the capability to sustain efficient operations over a wide temperature range. 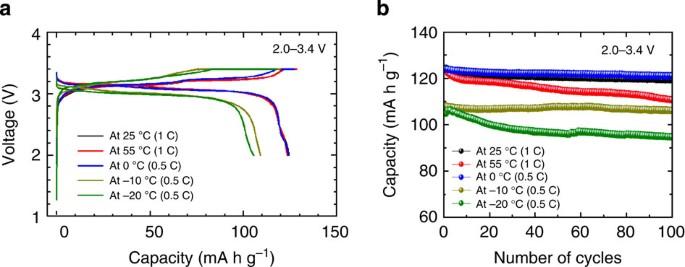Figure 6: Performance of the LTO/LNMO battery at various temperature. (a) Shows the voltage profiles of the charge-discharge cycles of the battery in a temperature range extending from −20 to +55 °C demonstrating excellent voltage and capacity retention. (b) Shows that even at these extreme temperature limits, the battery cycles with a very stable capacity delivery and at comparatively high rates. Figure 6a shows that the LTO/LNMO battery developed in this work fulfills this requirement as it cycles with excellent voltage and capacity retention over a temperature excursion spanning from −20 to +55 °C. In addition, even at these extreme temperature limits, the battery cycles with a very stable capacity delivery ( Fig. 6b ). Figure 6: Performance of the LTO/LNMO battery at various temperature. ( a ) Shows the voltage profiles of the charge-discharge cycles of the battery in a temperature range extending from −20 to +55 °C demonstrating excellent voltage and capacity retention. ( b ) Shows that even at these extreme temperature limits, the battery cycles with a very stable capacity delivery and at comparatively high rates. Full size image We are aware that the concept of combining LTO with different positive electrode materials to form stable and long-life batteries is not new. It was originally proposed in 2003 by Ohzuku and co-workers [19] and in 2004 by us [20] , and it is presently exploited in various laboratories [21] , [22] . With this work, we have marked a step forward in the field as the LTO/LNMO battery here reported shows rate, life and energy performance, to our knowledge, never reached before. From the data of Figure 5 , that demonstrate a stable capacity delivery of 124 mA h g −1 , a maximum value of 372 W h kg −1 of energy density is obtained. By using the accepted 40% penalty factor to account for the weight of the electrolyte and of the ancillary components (case, current collectors and so on), a practical energy density of 225 of W h kg −1 may be anticipated, that is, a value considerably higher than that delivered by the presently available Li-ion batteries. In addition, our LTO/LNMO battery, in virtue of the high tap density of the electrodes, is also expected to have a high volumetric energy density, estimated of the order of 540 W h l −1 . Last, but certainly not least, the unique morphology of the electrode consents the battery to operate at high rates over a temperature range extending from −20 to 55 °C. We believe that all the above stressed features make the LTO/LNMO battery here reported a unique electrochemical device that outclasses other competitor systems for operation in the energy and transportation fields. Synthesis of C-LTO The microscale, C-coated Li 4 Ti 5 O 12 anode material was prepared by mixing highly mesoporous anatase TiO 2 with a stoichiometric amount of Li 2 CO 3 and pitch as the carbon-coating source. The carbon content in C-Li 4 Ti 5 O 12 was 5.2 wt%. Details of the synthesis route are reported in previous papers [12] , [23] , [24] . The spherical Li[Ni 0.45 Co 0.1 Mn 1.45 ]O 4 cathode was synthesized by co-precipitation of NiSO 4 ·6H 2 O, CoSO 4 ·7H 2 O and MnSO 4 ·5H 2 O. Details of the preparation procedures are reported elsewhere [16] , [25] . Morphology and structure studies The morphology of the synthesized materials was analysed by field-emission scanning electron microscopy (JSM-6400, JEOL) and high-resolution transmission electron microscopy (JEM-2010, JEOL). The structure was determined by Powder X-ray diffraction, carried out using a Rigaku Rint-2000 with Cu Ka radiation. The diffraction data were obtained at 2 θ =10° to 80°, with a step size of 0.03°. Preparation of electrodes and cells The electrodes were prepared by mixing powders of the active materials, that is, Li[Ni 0.45 Co 0.1 Mn 1.45 ]O 4 and C-coated Li 4 Ti 5 O 12 , respectively, with carbon black and polyvinylidene fluoride (80:10:10) in N -methylpyrrolidinon. The obtained slurry was coated onto Al or Cu foils, respectively, and roll-pressed. The electrodes were then dried overnight at 120 °C in vacuum, before use. The initial electrochemical tests were done with a 2032 coin-type cell using Li metal as the anode. The capacities of the electrodes were referred to the electrode material as a whole, including the minor carbon coating content. The size of the Li[Ni 0.45 Co 0.1 Mn 1.45 ]O 4 -positive electrode is 3 cm×5 cm and that of the negative C-Li 4 Ti 5 O 12 , is 3.1 cm×5.1 cm. The weight of the two electrodes were 104.4 mg and 112.2 mg, respectively, so as to lead to a N/P (negative/positive) electrode ratio of 1.36 in the laminated-type cell. Preparation of the battery The LTO/LNMO battery was assembled by a laminated-type full cell, wrapped with an Al pouch. The battery was cathode limited. The electrolyte solution was 1.2 M LiPF 6 in ethylene carbonate-dimethyl carbonate (3:7 in volume). Battery tests The batteries were charged and discharged between 2.0–3.4 V voltage limits, at various C-rates (1 C rate corresponding to 135 mA h g −1 ) and at different temperatures. The PCGA test was performed using a VMP biologic-science instrument with a stepwise potential scans of 5 mV and minimum current limit of 10 μA within a 1.0–3.0 V versus Li potential limits. The test was run in a three-electrode cell where the working electrode sample was combined with a lithium foil used as reference and counter electrode. How to cite this article: Jung, H.-G. et al . A high-rate long-life Li 4 Ti 5 O 12 /Li[Ni 0.45 Co 0.1 Mn 1.45 ]O 4 lithium-ion battery. Nat. Commun. 2:516 doi: 10.1038/ncomms1527 (2011).